Supersensitive fingerprinting of explosives by chemically modified nanosensors arrays The capability to detect traces of explosives sensitively, selectively and rapidly could be of great benefit for applications relating to civilian national security and military needs. Here, we show that, when chemically modified in a multiplexed mode, nanoelectrical devices arrays enable the supersensitive discriminative detection of explosive species. The fingerprinting of explosives is achieved by pattern recognizing the inherent kinetics, and thermodynamics, of interaction between the chemically modified nanosensors array and the molecular analytes under test. This platform allows for the rapid detection of explosives, from air collected samples, down to the parts-per-quadrillion concentration range, and represents the first nanotechnology-inspired demonstration on the selective supersensitive detection of explosives, including the nitro- and peroxide-derivatives, on a single electronic platform. Furthermore, the ultrahigh sensitivity displayed by our platform may allow the remote detection of various explosives, a task unachieved by existing detection technologies. Numerous recent adverse events have led to an increased requirement for improving our ability to detect highly energetic chemicals, explosives, making their detection an issue of burning immediacy, and a major current challenge in terms of research and development. The capability to detect traces of these hazardous chemical species sensitively, selectively, accurately and rapidly could be of great benefit for applications relating to civilian national security and environmental monitoring. Unfortunately, the reliable detection of explosives still represents a challenging, and a largely unmet, arduous problem. This is mainly due to the requirement to sensitively and selectively detect, and quantify, traces of a broad variety of explosive species in any given encountered environment. This challenge is further exacerbated by the inherently low vapour pressures of most of these compounds [1] . For instance, trinitrotoluene, TNT, exhibits a vapour pressure of a few parts-per-billion at room temperature (1 p.p.b. corresponds to only one TNT molecule in 1 billion molecules of air), while the more powerful, and less volatile, explosives RDX (1,3,5-Trinitro-1,3,5-triazacyclohexane) and HMX (Octahydro-1,3,5,7-tetranitro-1,3,5,7-tetrazocine) stands at a few parts-per-trillion (p.p.t.) and part-per-quadrillion (p.p.q. ), respectively. This directly means that the detection system must be highly sensitive, while simultaneously exhibiting rapid response and high selectivity. Furthermore, the detection of improvised peroxide-based explosive species, that is, TATP (Triacetone triperoxide) and HMDT (Hexamethylene triperoxide diamine), is strongly challenged by the inherent absence of nitro groups and their poor spectroscopic features. Even though multiple strategies have been developed for the detection of explosive species [2] , [3] , [4] , these methods are usually time consuming, require bulky equipment, tedious sample preparation and a trained operator. Furthermore, these systems cannot be miniaturized and lack the ability to perform automated real-time high-throughput analysis, strongly handicapping their mass deployment. Due to their reduced dimensions, nanomaterials offer the ability of incorporating multiple sensors capable of detecting numerous chemical threats simultaneously on a single miniature array platform [5] , [6] , [7] . Thus, nanoscale device arrays have the potential to generate sensors with ultrahigh sensitivity, exceptional specificity towards a wide-range expandable ‘library’ of detectable threats, real-time unlabelled detection, samples versatility (gas, liquid and particles), and portable easily-operable devices. In general, 1D-nanowire building blocks, when configured as nanoFET (nano Field Effect Transistor) devices, are extremely sensitive to the absorption of chemical species on their surface, due to their intrinsically high surface-to-volume ratio, leading to significant changes in their resulting electrical conductance [8] , [9] , [10] , [11] , [12] . Traditionally, analyte detection relies on the specific chemical interactions between a ligand and its probe, entailing complexity, high costs and time consuming fabrication processes. Besides, a one probe-one ligand approach excludes the identification of not yet identified analytes. The growing interest to make use of such intriguing nanoscale building blocks for the detection of explosive species, has led to the recent application of chemically modified nanowire FETs as ultrasensitive label-free trace sensors for TNT molecules [13] , attaining an unprecedented limit of detection in the low femtomolar (p.p.q.) concentration range. Despite the exquisite achieved sensitivity, the use of nanodevices chemically modified with a single ‘unspecific’ molecular binding agent led to a strongly limited selectivity, and the consequent absolute inability to discriminate between the binding of explosive molecules and that of different, similar and dissimilar, chemical species [2] . Clearly, in order to make full advantage of nanosensing devices in the field of explosives detection, and other small molecular species, existing challenges related to sensitivity and selectivity must be jointly overcome. Inspired by nature, artificial sensing systems mimic the mammalian olfactory system, in which a finite number of not highly selective cross-reactive receptors generate a response pattern that is perceived by the brain as a particular odour. This general approach make use of a library of sensitive materials, the artificial cross-reactive sensors that differentially interact with the target molecules, and generates a fingerprinting pattern that is recognized by pattern-recognition chemometric tools [14] , [15] , [16] , [17] , [18] . Here, we present the development of an ultrasensitive and highly selective platform for the detection and discriminative identification of explosive chemical species, based on the use of large-scale arrays of chemically modified electrical nanosensors, defining a plurality of multiple functional reaction sites enabling a high-throughput assay. When chemically modified in a multiplexed mode, by the surface immobilization of multiple non-specific small chemical receptors, nanowire-based field-effect-transistor arrays (NW-FETs) enable the supersensitive discriminative detection, fingerprinting, of multiple explosive molecules, down to the parts-per-quadrillion concentration range [19] . The differential identification between explosives is achieved by pattern recognizing the naturally inherent interaction, both kinetically and thermodynamically [20] , [21] , [22] , [23] , [24] , [25] , [26] , [27] , between the chemically modified nanosensors array and the chemical analytes under test. Thus, a unique explosives fingerprinting database can be created, enabling to set apart similar chemical entities, and providing a fast and reliable method to identify individual chemical agents. This allows the direct detection of explosives species displaying the lowest volatilities, as well as the remote detection of various explosive species. The chemically modified nanosensors array The multiplexed high-throughput detection and identification of explosives by a single chip is achieved by fabricating a SiNW-FETs multiarray (144 FET devices per chip, functioning devices yield of 60–70%), containing eight subarrays in total, each subarray consisting of 18 FET nanodevices, being individually modified by a unique surface binding agent. All subarrays are fed by a common integrated microfluidic channel that enables the flow and interaction of all analytes with the modified array, Fig. 1a,b . p-type boron-doped silicon nanowires (p-type SiNWs) were grown by the vapour-liquid-solid chemical vapour deposition method, followed by dry transferring to their destined locations on chip, and the formation of electrical contacts by common lithography and metal deposition steps [13] , [28] , [29] . Metal source and drain contacts were passivated by a thin 60 nm silicon nitride layer, deposited using PECVD (plasma-enhanced chemical vapour deposition), which electrically isolates the metal electrodes from the sensing solution ( Supplementary Fig. 1A,B ). The resulting 144 nanosensor devices were electrically characterized and effectively normalized by their respective transconductance values, thus minimizing the device-to-device signal variability [30] , Fig. 2 . Using SiNWs as the sensing elements, various selected surface-bound electron-rich aminosilane derivatives chemically pair with the explosive molecules in a sample, by charge-transfer (e.g., Meisenheimer complexes) and additional chemical interactions [31] , thus leading to the formation of charges or surface dipole alteration, in close vicinity to the sensing surfaces. Since the analyte molecules are not of biological nature, salt-free baseline solution is used in all our sensing experiments (0.1% dimethyl sulfoxide (DMSO) in H 2 O), enabling electrolyte screening-free conditions, resulting in a large Debye length (~\n1 μm [21] , [32] ) that confers extremely high detection sensitivity. 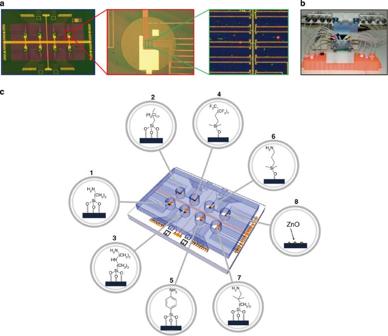Figure 1: View of the multiplex sensing chip. 144 NanoFET devices sharing a common liquid gate, arrayed into eight separate subregions, chemically modified with eight different chemical receptors. (a) Progressive magnifications of a sensing chip, wherein p-doped SiNWs channels, bridge a common source (middle electrode) with its surrounding drain electrodes. (b) Eight chemically differentiated subregions are created by simultaneously flowing different silane derivatives onto their designated pads, using a dedicated eight-channel fluidic device. (c) Scheme of a chip bearing eight chemically differentiated subregions. (1) Aminopropyltriethoxysilane (APTES), (2) N-Octadecyltriethoxysilane (OTS), (3) n-(2-aminoethyl)-3-3aminopropyltrimethoxysilane, (en-APTAS), (4) (Heptadecafluoro-1,1,2,2-tetrahydrodecyl)dimethylchlorosilane (Fluorosilane), (5) p-aminophenyltrimethoxysilane (p-APhS), (6) Aminopropyldimethylmethoxysilane (APDMES), (7) 4-amino-3,3-dimethylbutyl triethoxysilane (tBu), (8) silicon oxide, non-modified SiNW, or NPs-decorated devices. Figure 1: View of the multiplex sensing chip. 144 NanoFET devices sharing a common liquid gate, arrayed into eight separate subregions, chemically modified with eight different chemical receptors. ( a ) Progressive magnifications of a sensing chip, wherein p-doped SiNWs channels, bridge a common source (middle electrode) with its surrounding drain electrodes. ( b ) Eight chemically differentiated subregions are created by simultaneously flowing different silane derivatives onto their designated pads, using a dedicated eight-channel fluidic device. ( c ) Scheme of a chip bearing eight chemically differentiated subregions. ( 1 ) Aminopropyltriethoxysilane (APTES), ( 2 ) N-Octadecyltriethoxysilane (OTS), ( 3 ) n-(2-aminoethyl)-3-3aminopropyltrimethoxysilane, (en-APTAS), ( 4 ) (Heptadecafluoro-1,1,2,2-tetrahydrodecyl)dimethylchlorosilane (Fluorosilane), ( 5 ) p-aminophenyltrimethoxysilane (p-APhS), ( 6 ) Aminopropyldimethylmethoxysilane (APDMES), ( 7 ) 4-amino-3,3-dimethylbutyl triethoxysilane (tBu), ( 8 ) silicon oxide, non-modified SiNW, or NPs-decorated devices. 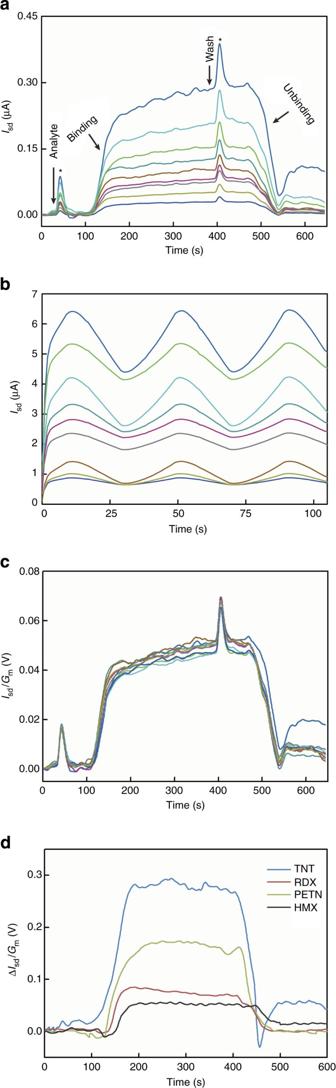Figure 2: Signal processing steps. (a) The raw sensing response to TNT over time of nine APTES-modified active sensing devices. (*) two peak rises at 50 s and 400 s are caused by a pinch valve pressure artifact. (b) The transconductance response of the same sensing devices as a function of the gate voltage (time at a given scan rate) being periodically modulated between −0.3 V and +0.3 V. (c) Calibrated responses of devices ina, after normalizing each device raw response by its gate dependence. After calibration, all nine devices display almost identical electrical behaviour. (d) Calibrated responses of a representative APTES-modified nano FET device to different explosive species at the same concentration, 10 p.p.t., displaying the inherent lack of selectivity. Full size image Figure 2: Signal processing steps. ( a ) The raw sensing response to TNT over time of nine APTES-modified active sensing devices. (*) two peak rises at 50 s and 400 s are caused by a pinch valve pressure artifact. ( b ) The transconductance response of the same sensing devices as a function of the gate voltage (time at a given scan rate) being periodically modulated between −0.3 V and +0.3 V. ( c ) Calibrated responses of devices in a , after normalizing each device raw response by its gate dependence . After calibration, all nine devices display almost identical electrical behaviour. ( d ) Calibrated responses of a representative APTES-modified nano FET device to different explosive species at the same concentration, 10 p.p.t., displaying the inherent lack of selectivity. Full size image Up to eight different surface-confined chemical receptors, molecules 1 to 8 ( Fig. 1c ), were selectively anchored to separate nanosensors subarray spots, each subarray containing 18 devices, by the use of area-selected silane-coupling procedures [33] , [34] , [35] , as schematically depicted in Fig. 1 ( Supplementary Figs 2 and 3 ). The successful modification of the different silane derivatives was characterized by XPS measurements (X-ray photoelectron spectroscopy; see Methods and Supplementary Methods Sections for experimental details and data). The surface coverage of the different silane derivatives was measured by means of QCM (quartz crystal microbalance) measurements (see Methods for details), and strongly depends on the chemical nature of the silane derivative molecule. Polar silanes display lower surface coverage, in the order of ~\n3–6 × 10 13 molecules˙cm −2 , while non-polar derivatives display higher surface coverage of ~\n1–4 × 10 14 molecules˙cm −2 . The silanes layers were demonstrated to be highly stable for periods of weeks of continuous operation under our experimental conditions. Generally, the interaction of electron-deficient nitro-containing explosives with amine groups of silane receptor molecules leads to the formation of surface-confined charges [36] , [37] , consequently alterating the nanodevices electrical response. During the measurements, differential gating can be applied at the subthreshold or threshold regimes [38] , while the applied V SD bias (source-drain voltage) allows operation at a particular region of the device's transconductance. The detection of explosives by nanosensors array All our sensing experiments using nanoFETs arrays are performed in liquid phase, in a solution of 0.1% DMSO in H 2 O, as stated in the manuscript body and methods section. All sensor calibrations, detection limits extraction, kinetic and thermodynamic parameters measurements and real-world tests, are done in the liquid phase using explosive standard solutions (purchased from AccuStandard Inc.). When collecting explosives’ vapours off the air, the analyte molecules are partitioned onto a solid surface whence they are washed off with the sensing solution collected and tested. In practice, the detection of real-world samples is separated into two sequential steps, performed automatically by our sensing prototype, where the air sample is collected for 5 s through a micro-porous filter support by means of an air sampling device (sampling of 50–100 l min −1 ), then the adsorbed analytes are flushed off the collecting membrane by the sensing solution, and finally channelled into the sensing area for detection. The resulting change in the source-drain current ( I SD ) that flows through the chemically modified nanodevices is a function of the change in the chemical and electronic environment. Thus, when target molecules in the sample attach to the nanodevices’ surface, a change occurs in their conductance–resulting in a change in the measured current and indicating the detection of the target molecule. Figure 2a displays the electrical shifts observed upon the interaction of several nanodevices on a single chip, modified with the amine-containing receptor APTES (aminopropyl triethoxy silane) (1) , with TNT-containing samples. The devices are real-time sensors, and quickly regenerate after each sensing cycle by flushing a pulse of washing solution that restores the devices to their initial baseline. Hundreds of sensing cycles can be performed using a single sensing platform, for periods of weeks, without considerable degradation of the detection performance. Notably, the whole detection cycle, from explosive sample injection till final detection (binding, plateau, unbinding), can be speeded up down to ~\n30 s, Supplementary Fig. 4 . Clearly, the calibrated responses of the devices to the analyte (Δ I sd ), when normalized by their respective transconductance values (device transconductance ), Fig. 2b , will result in relatively small device-to-device variability, even for originally largely dissimilar devices [30] , Fig. 2c . Furthermore, a large number of sensors allows redundancy, thus improving the signal-to-noise ratio, and offers the ability to reject the output of poorly performing sensing devices [15] . Moreover, the reproducibility displayed by a single FET sensor to the repeated interaction with a certain explosive is remarkable, Supplementary Fig. 4A–D . Clearly, the single-sensor sequential responses display a remarkable level of reproducibility, both regarding their signal plateau (thermodynamically, values of Δ G from baseline to peak) as well as regarding the complex kinetics responses. Of, course, the same behaviour is observed for all devices in a single array, regardless their chemical modifier and location on the array. These results show the ability of our platform, to identify different molecular species with a high level of reliability and reproducibility. Importantly, all devices modified with molecular receptor APTES (1), also show considerable electrical shifts and cross-reactivity, upon their interaction with different explosive species at concentration of 10 p.p.t. : TNT, RDX, HMX and PETN ([3-Nitroxy-2,2-bis(nitromethyl)propyl]nitrate), Fig. 2d , as well as upon their interaction with non-explosive interferents (for example, Ammonium Nitrate, Musk ketone, Musk moskene). Although the interaction with the highly electron-deficient TNT molecules leads to the largest measured electrical shifts, with detection limits down to the p.p.q. (parts-per-quadrillion) concentration range, these results show the complete incapability to selectively detect different explosive species by nanodevices chemically modified with a single molecular receptor, regardless the chemical receptor used for detection, as per previously reported cases [13] . The discriminative identification of explosive species A potential advantageous approach for the selective detection of explosives, and their discriminative identification, is based on the real-time mathematical analysis of their interaction, both kinetically and thermodynamically, with a single array bearing multiple molecular binding agents. To that end we have tested a broad library of aminosilane derivatives for their interaction with multiple explosive species of relevance. Our selected surface-confined binding agents ( Fig. 1c ) consist of primary amines (APTES, en-APTAS 3-(2-Aminoethylamino)propyltrimethoxysilane, tBu (4-amino-3,3-dimethylbutyl triethoxysilane), APDMES (3-aminopropyl)-dimethyl-ethoxysilane), secondary amines (en-APTAS), aromatic amines (aniline derivatives m-APhS (aminophenyl triethoxy silane) and p-APhS), as well as amine-free silane derivatives (OTS (octadecyltrichloro silane), fluorosilane derivatives), serving as control explosives-non-binding compounds ( Supplementary Table 1 ). Clearly, each type of aminosilane modifier has different chemical, steric and electronic characteristics. Our nanoarray chip, with integrated multichannel microfluidics, allows for the differential yet simultaneous chemical modification of all eight subarrays with multiple surface binding agents, as illustrated in Fig. 1b . Generally, 1% ethanolic solutions of each silane derivative are simultaneously and separately flowed along their respective wells, by means of individual inlet and outlet ports, followed by washing the unbound silanes excess before the final curing step (see Methods for detailed information and Supplementary Figs 2 and 3 ). In this case, each explosive species is expected to exhibit a distinctive pattern of interaction, both kinetically and thermodynamically, with the chemically modified nanodevice array. For that purpose, Fig. 3c , we chose to make use of two parameters inherent to the interaction between any explosive chemical species and the surface-confined chemical receptors: (1) the signal amplitude, or electrical shift, measured after reaching the asymptotic saturation value of the device ( I sd after equilibrium is achieved) at any concentration of the given explosive, when the Δ I sd was calibrated by its gate dependence, the transconductance value ( G m ), and (2) the initial rates of association, and dissociation, measured after the interaction of the array with a certain explosive species, and the sequential flushing of the sensors surface with a clean baseline solution leading to the unbinding of the explosive species, V 1 and V 2 respectively. To achieve this goal, we developed a five-tier algorithm (for more information see Supplementary Methods ) able to extract, and analyse, in real time all the above mentioned parameters, Fig. 3a–e , followed by the final identification of the molecular species under test based on a formerly built fingerprints database Fig. 3e (see Supplementary Methods ). 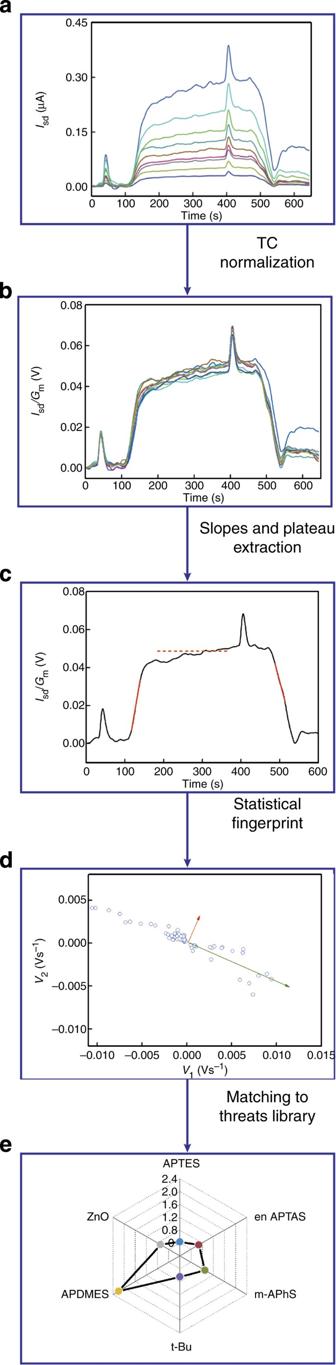Figure 3: Signal processing algorithm steps. Raw response (a), followed by calibrating each device’s absolute raw electrical response against its gate dependence(b). Mathematically extracting the following parameters: the kinetic ratio (V1/V2) and the calibrated absolute response under steady state conditions, at plateau (c). Data processing ensues, whereby the statistical dependence of the kinetic constants is globally estimated by the slope of a straight line in theV1–V2plane obtained by regression usingR2as a target function, taking into account all accumulatedV1–V2pairs (d). Chemical identification, wherein a matching is done between the pattern generated by the given ensemble response and a library of previously calculated responses (e). Figure 3: Signal processing algorithm steps. Raw response ( a ), followed by calibrating each device’s absolute raw electrical response against its gate dependence ( b ). Mathematically extracting the following parameters: the kinetic ratio ( V 1 /V 2 ) and the calibrated absolute response under steady state conditions, at plateau ( c ). Data processing ensues, whereby the statistical dependence of the kinetic constants is globally estimated by the slope of a straight line in the V 1 – V 2 plane obtained by regression using R 2 as a target function, taking into account all accumulated V 1 – V 2 pairs ( d ). Chemical identification, wherein a matching is done between the pattern generated by the given ensemble response and a library of previously calculated responses ( e ). 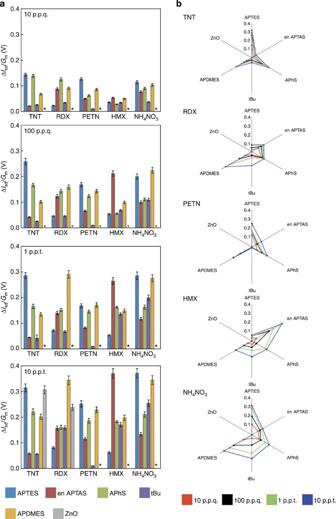Figure 4: Thermodynamics-based analysis. (a) At a steady state, the calibrated absolute response of different silanes to a certain explosive species is discriminative, such that their relative responses create a concentration-independent pattern to make an explosive’s unique fingerprint. (1) Aminopropyl triethoxysilane (APTES), (3) n-(2-aminoethyl)-3-3aminopropyltrimethoxysilane, (en-APTAS), (5) p-aminophenyltrimethoxysilane (p-APhS), (6) Aminopropyldimethylmethoxysilane (APDMES), (7) 4-amino-3,3-dimethylbutyl triethoxysilane (tBu), (8) ZnO NPs-decorated devices, against different explosives (TNT, RDX, HMX, PETN and NH4NO3). Errors bars represent the measured values range forn>50 measurements. Asterisks denote the absence of electrical response of the nanodevice upon interaction with the respective explosive. (b) The ‘radar plot’ two-dimensional presentation for the interaction of each explosive species with six different surface receptors, at different concentrations. The radar plots of each explosive at different concentrations are overlapped in order to demonstrate the concentration independency of our fingerprinting approach. Full size image Figure 4a,b displays the results obtained from the interaction of several common explosives with a multireceptor array of nanosensors modified with molecular receptors ( 1 , 3 , 5 , 6 , 7 and 8 of Fig. 1c ). Explosives samples were obtained by collecting air samples of explosives-containing solid sources, at room temperature, on filter supports (by short sampling pulses of 5 s). Alternatively, calibrated standard solutions containing known concentrations of the respective explosives were prepared and flowed into the sensing system. Figure 4a,b presents the interaction of each explosive species, in terms of Δ I sd / G m values measured under steady state conditions, (constant analyte concentration under constant flow) with various molecular binding receptors of the chemically modified nanoarray. Clearly, different explosives species display a distinctive pattern of interaction with the nanosensing array, thus allowing for a simple and straightforward identification of the molecule under test. The interaction pattern of each explosive species is kept constant regardless its concentration in the tested sample, Fig. 4b . Notably, all devices display a clear concentration-dependent behaviour when exposed to different concentrations of a certain explosive species, Supplementary Fig. 5a,b . Also, this distinctive fingerprinting pattern of interaction is common to all devices within a single nanoarray platform (for all the eight subarrays of 18 nanoFETs each), and across different nanoarray chips ( n >100 chips). Furthermore, control unmodified nanodevices on the same chip, as well as devices modified with non-amino silanes (for example, alkyl or fluoroalkyl silanes) do not produce any observable signal upon interacting with even relatively high concentrations of explosives (in the high μM range, hundreds of p.p.m. level, confirming previous reports [13] , [21] ). Importantly, these devices demonstrate the need for electron-donating functional groups, for example, amine, thiol groups [9] , [39] and possibly calyx[4]pyrrole receptors [40] , required for the binding interaction of the electron-deficient explosive species to the nanosensors surface, and thus will be applied as the internal control sensors throughout our studies. Figure 4: Thermodynamics-based analysis. ( a ) At a steady state, the calibrated absolute response of different silanes to a certain explosive species is discriminative, such that their relative responses create a concentration-independent pattern to make an explosive’s unique fingerprint. ( 1 ) Aminopropyl triethoxysilane (APTES), ( 3 ) n-(2-aminoethyl)-3-3aminopropyltrimethoxysilane, (en-APTAS), ( 5 ) p-aminophenyltrimethoxysilane (p-APhS), ( 6 ) Aminopropyldimethylmethoxysilane (APDMES), ( 7 ) 4-amino-3,3-dimethylbutyl triethoxysilane (tBu), ( 8 ) ZnO NPs-decorated devices, against different explosives (TNT, RDX, HMX, PETN and NH 4 NO 3 ). Errors bars represent the measured values range for n >50 measurements. Asterisks denote the absence of electrical response of the nanodevice upon interaction with the respective explosive. ( b ) The ‘radar plot’ two-dimensional presentation for the interaction of each explosive species with six different surface receptors, at different concentrations. The radar plots of each explosive at different concentrations are overlapped in order to demonstrate the concentration independency of our fingerprinting approach. Full size image In addition, kinetic parameters inherent to the chemical interaction between different explosives species and the chemically modified nanosensors array can be simultaneously extracted and analysed, together with thermodynamic parameters, to enhance the selectivity of the sensing process, and the accurate identification of the molecular species under test. The ‘kinetic parameters’ referred in this work are the initial slopes, the very first seconds, of the reactions that occur between the explosive species and surface-confined binding receptors. In other words, after each explosive binds and unbinds, the initial slopes of I SD as a function of time indicate the binding ( V 1 ) and unbinding ( V 2 ) processes, respectively. After measuring V 1 and V 2 , the kinetic factors of six silane-based receptors against different explosive species, as per Figs 4 and 5 , are calculated. The kinetic data is summarized in Fig. 5a,b . Significantly, every silane-to-explosive couple has its own and unique kinetic V 1 /V 2 ratio, creating together a kinetic data matrix. This matrix is actually a library–or ‘fingerprint’–of each one of the explosives under measurement; of course, measuring additional materials (both explosives and silanes) will expand this database and will enable us to update it, and enable the detection and identification of novel types of explosives. Note that our measurements of the kinetics complex ratios of any given explosive species with the chemically modified array do not show a concentration-dependence behaviour (in the range of 1 p.p.q.-1 p.p.b. ), but only affected by the nature of the explosive-to-receptor pair under investigation. Notably, potential interfering molecules will give rise to considerably different interaction patterns with the chemically modified nanosensors array, and may be easily discriminated in real-time from known explosive molecules of interest. In addition, by virtue of our developed algorithm, and the multiplexed nature of the sensing array, we are capable of detecting and identifying explosives mixtures ( Supplementary Fig. 6 ), interfering species and taggant species ( Supplementary Fig. 7 ). Furthermore, the multiparameter combined use of kinetics- and thermodynamics-based analyses, Figs 4 and 5 , allows for a more accurate and clear-cut identification of the molecular species under test, as described in Fig. 6 . Figure 6 practically exemplifies the complete set of results obtained when exposing the multireceptor nanosensor array to a certain explosive sample. 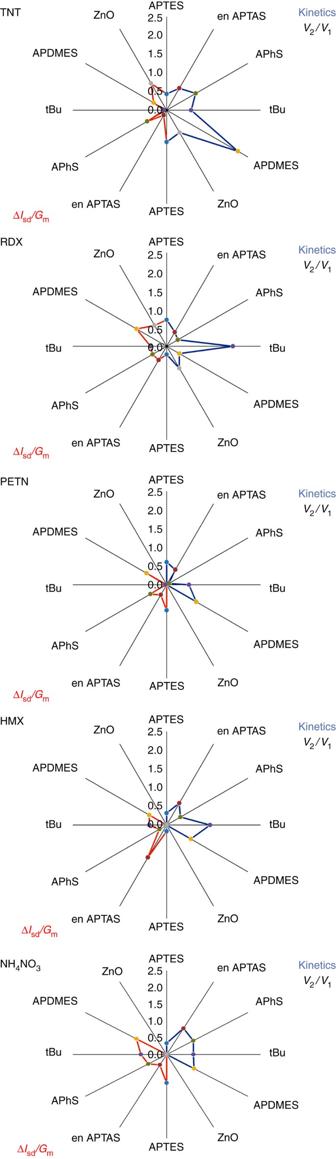Figure 6: Fingerprinting explosives by combining kinetics and thermodynamics. The algorithm-derived analysis results of the interaction of the multireceptor sensor platform (consisting of1,3,5,6,7and8) after its exposure against various explosive species, combining the results separately described inFigs 4and5. Left side ΔG/Gmaxrepresents the thermodynamic-derived results for each explosive (red colour), and the right side represents the kinetics-derived results for each explosive species (blue colour). Furthermore, in order to show the selectivity and relative insensitivity of our sensing platform to potentially interfering environments, we have carried out experiments for the detection of explosives under highly contaminated conditions, for example, cigarette-smoke heavily polluted air samples. Supplementary Fig. 8 demonstrates the capability to detect a sample of 10 p.p.t. TNT on a series of APTES-modified nanoFET devices away from smoke-highly contaminated samples. 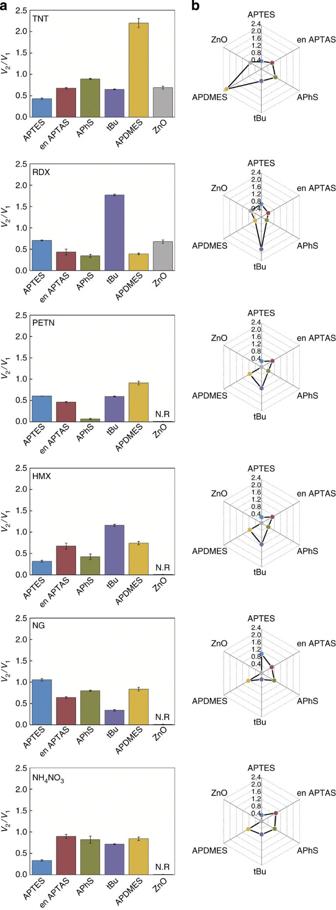The direct 30 s collection of air samples from a lighted cigarette, by the air sampling device through a filter support, does not cause any electrical responses on the sensor devices, while a 5 s air collection of TNT vapour samples (from above a solid TNT source) leads to clear-cut electrical responses from all FET devices. Figure 5: Kinetics-based analysis. (a) The algorithm-derived kinetic ratios of the real-time measured transient electrical signals (V1–V2) map. Multiple explosive species are tested against the silanes-modified sensing array, to create a unique fingerprint pattern that enables the discrimination of all tested explosives (see ‘radar’ two-dimensional presentation on panel (b)). The whole set of mathematically derived kinetics produces a profile library (left panel, bar graph), where each result is calculated over >50 experiments performed with at least five different chips. (APTES, Aminopropyltriethoxysilane; en-APTAS, n-(2-aminoethyl)-3-3aminopropyltrimethoxysilane; p-APhS, m-aminophenyltrimethoxysilane; APDMES, Aminopropyldimethylmethoxysilane; tBu, 4-amino-3,3-dimethylbuthyltriethoxysilane; ZnO, zinc oxide-decorated SiNWs). Errors bars represent the measured values range forn>50 measurements. Figure 5: Kinetics-based analysis. ( a ) The algorithm-derived kinetic ratios of the real-time measured transient electrical signals ( V 1 – V 2 ) map. Multiple explosive species are tested against the silanes-modified sensing array, to create a unique fingerprint pattern that enables the discrimination of all tested explosives (see ‘radar’ two-dimensional presentation on panel ( b )). The whole set of mathematically derived kinetics produces a profile library (left panel, bar graph), where each result is calculated over >50 experiments performed with at least five different chips. (APTES, Aminopropyltriethoxysilane; en-APTAS, n-(2-aminoethyl)-3-3aminopropyltrimethoxysilane; p-APhS, m-aminophenyltrimethoxysilane; APDMES, Aminopropyldimethylmethoxysilane; tBu, 4-amino-3,3-dimethylbuthyltriethoxysilane; ZnO, zinc oxide-decorated SiNWs). Errors bars represent the measured values range for n >50 measurements. Full size image Figure 6: Fingerprinting explosives by combining kinetics and thermodynamics. The algorithm-derived analysis results of the interaction of the multireceptor sensor platform (consisting of 1 , 3 , 5 , 6 , 7 and 8 ) after its exposure against various explosive species, combining the results separately described in Figs 4 and 5 . Left side Δ G / G max represents the thermodynamic-derived results for each explosive (red colour), and the right side represents the kinetics-derived results for each explosive species (blue colour). Full size image Detecting peroxide-based explosives on a single platform Lastly, but not of lesser importance, is our capability to directly and sensitively detect and identify peroxide-based explosives, such as Triacetone trioxide (TATP) and HMDT, infamous for their clandestine production due to the availability of the ingredients and the ease of production [41] . Conventional explosives sensors rely on the presence of nitro groups. Unlike conventional nitro-containing explosives, TATP displays a significant vapour pressure at ambient temperature (6.95 Pa at 25 °C [42] ), but because of the fact that it does not contain nitro groups, its detection poses a serious challenge [43] . HMTD further exacerbates this limitation by displaying an extremely low vapour pressure. Thus, the development of novel approaches for the sensitive and rapid detection of these hazardous molecules is of great importance in the field of homeland security. Unfortunately, peroxide-based explosives do not show any appreciable interaction with the chemically modified nanosensors array, modified with silanes 1 – 8 ( Figs 7c and 1c ), and even at the highest tested concentrations of tens of p.p.m. (part-per-millions). In order to overcome this limitation, we developed a strategy for the area-selected decoration of nanowire devices with ZnO nanoparticles, by a low-temperature ALD (atomic layer deposition) process [44] . The area-selected decoration of ZnO NPs is allowed by an additional photolithography masking step, before the subsequent chemical modification of the undecorated array areas with the silane derivatives can be performed, Fig. 7a . The decoration process leads to the formation of a dense layer of ZnO NPs on the NWs sensing elements, with the capability of controlling over the nanoparticles dimensions, between 4–10 nm, Fig. 7b . In addition, the same ALD-based process can be readily applied for the decoration of nanowire sensing elements with TiO 2 and In 2 O 3 nanoparticles. The deposited metal oxide nanoparticles will serve as a basis for the complexation and further detection of this challenging explosives family. Past theoretical studies have shown a plausible approach based on the formation of complexes between the molecular ring structures of these explosives and a central metal moiety, analogous to clatherates and crown ethers that selectively bind to ionic species in solution. These studies have predicted that TATP molecules can bind to several ions of different valency, with In 3+ , Zn 2+ and Ti 4+ showing the highest binding energy [45] . On the basis of these studies, we confidently assumed that surface-decorated metal oxide nanoparticles will serve as effective complexating centres for the binding and detection of TATP and HMDT. Accordingly, Fig. 7d shows the interaction of ZnO NPs-decorated nanosensing devices in the presence of TATP, HMTD (Hexamethylene triperoxidediamine), TNT, RDX, PETN and HMX. These devices can sensitively detect TATP and HMTD down to the low p.p.t. concentration range, and effectively discriminate and identify these molecular species against all the nitro-containing explosives species tested before, Figs 4 , 5 , 6 , by the simple use of a single chemically modified sensing platform. Although TNT and RDX are sensed by the ZnO-decorated devices, they can only be detected at high concentrations of >100 p.p.t., and can be still easily discriminated by the complete thermodynamic and kinetic fingerprinting pattern extracted from their interaction with the multireceptor platform. As well, a clear discrimination, kinetically and thermodynamically, against simple peroxide species, that is, hydrogen peroxide, can be readily attained. 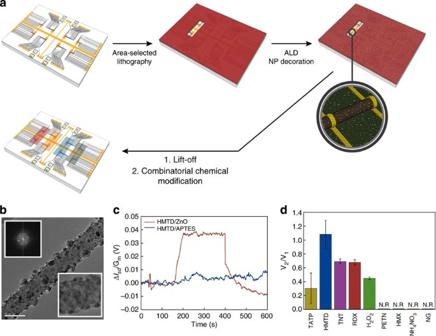Figure 7: Peroxides-based explosives detection. Peroxide-based explosives (TATP, HMTD) are detected by their unique complexation with zinc oxide nanoparticles decorating silicon nanowires (ZnO-SiNW). (a) Area-selected sensing regions are created on a multiplex chip by the ALD-assisted decoration of Si nanoFETs with ZnO nanoparticles, followed by resist removal to lay bare other subregions, to be in turn, chemically modified selectively with silane derivative receptors, as described inFig. 1. (b) Representative transmission electron microscopy image of ALD-deposited zinc oxide nanoparticles (70 °C, 10 cycles) decorating p-type SiNWs (~\n20 nm diameter). (c) Receptors that are sensitive to the nitro-carrying explosives family are mostly insensitive to the peroxide-based explosives family. The HMTD concentration is 1 p.p.t. (d) Besides peroxide-based explosives, ZnO complexes with TNT and RDX, yet is inert to HMX and the linear structured nitro-carrying explosives (PETN, NG). ZnO is known to donate electrons to H2O2, but hydrogen peroxide is detected only at high concentrations above 250 p.p.m. Irrespective of their concentration, all explosives are discriminated through their respective kinetic ratios. Errors bars represent the measured values range forn>50 measurements. Figure 7: Peroxides-based explosives detection. Peroxide-based explosives (TATP, HMTD) are detected by their unique complexation with zinc oxide nanoparticles decorating silicon nanowires (ZnO-SiNW). ( a ) Area-selected sensing regions are created on a multiplex chip by the ALD-assisted decoration of Si nanoFETs with ZnO nanoparticles, followed by resist removal to lay bare other subregions, to be in turn, chemically modified selectively with silane derivative receptors, as described in Fig. 1 . ( b ) Representative transmission electron microscopy image of ALD-deposited zinc oxide nanoparticles (70 °C, 10 cycles) decorating p-type SiNWs (~\n20 nm diameter). ( c ) Receptors that are sensitive to the nitro-carrying explosives family are mostly insensitive to the peroxide-based explosives family. The HMTD concentration is 1 p.p.t. ( d ) Besides peroxide-based explosives, ZnO complexes with TNT and RDX, yet is inert to HMX and the linear structured nitro-carrying explosives (PETN, NG). ZnO is known to donate electrons to H 2 O 2 , but hydrogen peroxide is detected only at high concentrations above 250 p.p.m. Irrespective of their concentration, all explosives are discriminated through their respective kinetic ratios. Errors bars represent the measured values range for n >50 measurements. Full size image Last but not least, the ultrahigh sensitivity attained by our nanosensing devices, in the low p.p.q. level, may allow the remote detection of various explosives species, without the need for physically contacting and collecting explosives’ trace particles, as commony practiced by current sensitivity-challenged devices. In this context, we have performed a broad series of real-world sensing experiments for the detection of ultra-low vapour traces of explosives, done by the collection of short pulses of air samples above solid sources of different explosives, as well as at different distances from these explosives sources (see Supplementary Note 1 and Supplementary Table 2 ). Our preliminary tests, have clearly shown the capability to detect the volatile TATP explosive at distances of at least 5 m from the solid open source. Also, the less volatile TNT explosive can be readily detected and discriminated from distances of up to 4 m from the explosive solid source. These results are in accordance with the remarkable sensitivity of our sensors, as well as with the calculated concentration-to-distance curves extracted for these explosives (see Supplementary Notes Section for detailed information on discussed results and calculations) [46] . These promising results demonstrate the potential capability of our sensing platform for the remote detection of explosive species. In conclusion, we have demonstrated the development of a chemically modified nanosensors array sensing platform for the supersensitive detection and identification of a broad range of chemically dissimilar explosive species. Besides its intrinsically unprecedented sensitivity, down to the low p.p.q. concentration range in gas and aqueous samples, the presented approach allows for the clear-cut discriminative identification of multiple explosives species based on the novel application of a real-time mathematical analysis, kinetically and thermodynamically, of the measured chemical interaction curves between the molecules under test and the individual surface-confined molecular receptors on the nanosensing elements. This analysis results in a clear fingerprinting of individual explosives molecules, and allows their identification and discrimination from non-explosives potential interferents. Furthermore, the sensitive rapid detection of peroxide-based improvised explosive species, TATP and HMTD can be performed by the decoration of nanosensing elements with metal oxide nanoparticles, e.g., ZnO, instead of the conventional surface modification by molecular silane derivatives. By means of a simple area-selected lithography procedure, we have demonstrated for the first time the fabrication of multiplexed sensing arrays consisting of molecularly-modified, as well as NP-decorated, nanosensing devices altogether in a single detection platform. In addition, the capability of this platform to remotely detect various explosive species was preliminarily demonstrated. We believe that these solid practical results represents the first generation of supersensitive, rapid and real-time analytical platform for the ultra-trace detection and identification of a broad range of explosives species. Undoubtedly, this approach can be naturally extended to the detection of additional small molecular and biomolecular species of interest. Materials and chemicals All silanes are products of Gelest Inc. (Morrisville, PA). All explosives are products of AccuStandard (New Haven, CT), NH 4 NO 3 from Sigma-Aldrich, Israel, while Musk moskene, Musk ketone and Musk xylene are from Fluka (Germany). Standard solutions of the explosives TNT, RDX, HMX PETN (1 part per thousand) are provided in methanol–acetonitrile 1:1mixtures, while HMTD, TATP (0.1 p.p.t.h) are solubilized in acetonitrile alone. All explosives, ammonium nitrate and the musk derivatives are solubilized and diluted in 0.1% DMSO (Sigma, Israel) solution in pure deionized water, 18.4 MΩ. Dimethyl Zinc and titanium isopropoxide ALD precursors, for the decoration of nanowire devices, were purchased from Sigma-Aldrich and used as received. AuNPs (20 nm) from BBI International (UK), and poly-L-lysine from Ted Pella Inc. (Redding Ca). SiH 4 gas 99.9999%, high-purity Argon 99.9999%, and diborane were purchased from Linde Germany. Three inch 600 nm thermal oxide-covered p-type <100> silicon wafers were supplied by Silicon Quest International (Reno, NV). LOR-5A copolymer and S-1805 photoresist were purchased from MicroChem Corp. Analytical-grade toluene was purchased from Frutarom, Israel. Experimental procedures SiNW growth is described in detail elsewhere [29] . Briefly, all NWs used in this work were grown by the VLS technique, using high-purity silane (SiH 4 ), high-purity argon as a carrier gas and 20 nm AuNPs serving as catalysts adhered to the growth substrate by a layer of poly-L-lysine. Nanowires were doped in situ with diborane, leading to 1:4,000 (B:Si ratio) p-type nanowire elements. The resultant crystalline NWs, with a final diameter of ca . 20 nm and ca . 10–20 microns long, exhibit a smooth surface with a thin native silicon oxide layer ( ca . 2 nm), as confirmed by transmission electron microscopy. Nanowire-based FETs array fabrication The Si wafers were cleaned by washing with acetone, isopropyl alcohol (IPA), DIW, incubation in hot Piranha for 5 min, rinsing thoroughly with deionized water (DIW), blowing with dry N 2 followed by oxygen plasma treatment (100 W, 50 sccm O 2 for 200 s (Axic HP-8 USA)). Source and drain electrodes were defined by mask exposure of a multilayer resist structure consisting of 500 nm LOR-5A copolymer and 500 nm S-1805 photoresist (purchased from MicroChem Corp.). After exposure, development and gold metallization of the gate, drain and source electrodes pattern (VST Israel), SiNWs were arrayed on their respective eight pads by a dry transfer method, as published in past [47] . Briefly, a lab-built contact printer brought together the opposing surfaces of the SiNWs donor surface and the chip aligned in such a way that the SiNWs would be transferred onto their destined 8 pads, with the NWs aligned perpendicularly to the surface of each source and its respective drain. A pressure of 10 g cm −2 was applied, at a constant velocity of 10 mm min −1 , for a distance of 10 mm. To eliminate all redundant NWs, except those destined to be channels at the active eight pads, a protecting mask of a resist pattern was created and the chip was treated by DRIE (PlasmaTherm, USA) under the following conditions: C 4 F 8 (10 sccm), SF 6 (50 sccm), RF1 (bias) 100 W, P =5 mTorr and t =13.5 s followed by incubation at PG remover (15 min, 70 °C), wash with acetone and IPA. The drain electrodes were defined, developed and metalized by e-beam evaporation of Ti/Pd/Ti (5/60/10 nm), respectively (VST Israel), and then passivated with an insulating dielectric layer of Si 3 N 4 (50 nm-thick) deposited by Inductively Coupled Plasma-Enhanced Chemical Vapour Deposition (ICP-PECVD) (Axic, USA). To eliminate the creation of analytes depots on the chip that might affect the measured results, the chip was protected from the environment by SU8, except the active pads areas. Open pads were defined by photolithography using negative photoresist, SU8 2000.5, spin coated at 500 r.p.m. for 10 s and at 3,000 r.p.m. for 30 s, to achieve a layer of ~\n500 nm thickness, followed by a pre-baking step (95 °C for 1 min). Photolithography is done at 350–430 nm, with an exposure time of 7 s, using a lithography mask ( Supplementary Fig. 1 ), followed by post-baking step (95 °C; 1 min) and development (1 min) and finally, IPA wash (10 s), and drying with N 2 . The wafer was hard baked at 150 °C for 15 min. Atomic layer deposition (Savannah 200 Cambridge Nanotech, Waltham, MA) was used to grow Zinc oxide nanoparticles (ZnO or TiO 2 NPs) over SiNWs located on their destined exposed pads (70 °C, 10 cycles, each cycle having the following sequence: H 2 O 0.015 s, wait 5 s, dimethyl zinc (or titanium isopropoxide) 0.015 s, wait 10 s. Devices electrical characterization IV measurements were taken for each device using a probe station (Janis Research Co., Washington) at room temperature. (1) The drain current ( I ds ) response to the applied V ds , varying between −0.3 V to +0.3 V at 10 mV s −1 rate, at constant gate bias (taken from +0.4 V to −0.4 V). The gate dependence of the device was established by taking the drain current I DS response in time for varying V g from −0.3 V to +0.3 V at 10 mV s −1 rate, at a constant V DS bias (0.1 V). The transconductance ( g m ) is given by the slope of I ds − V g at the linear section. Since the separation between the source and drain electrodes dictates a channel length of 3 μm and because the dry transfer aligns the SiNWs perpendicular to the electrode’s surface, we confidently conclude that the g m need not to be corrected since the length of the active channel is constant. Surface modification of a multiplex chip Silane surface modification is performed as follows: The cleaned chip is dried over a hotplate (115 °C, 1 h) and fitted over with a multiple ports flow through PDMS microfluidic system (plasma treated first (30 W, 50sccm O 2 , 3 min)) that enables the surface modification of the chip with several silanes simultaneously ( Supplementary Fig. 3 ). All silane solutions are made of 1% silane (v/v) in 95%: 5% mixture of ethanol with water adjusted to pH=5 (with glacial acetic acid), while heptadecafluoro-1,1,2,2, is modified in 2% silane solutions of 95% ethanol/DIW and 1:1dichloromethane/heptane. All mixtures are incubated for 20 min at RT and filtered through a 0.2 μm-cutoff. Silanes are infused through the microfluidic device over their destined pads at 3 μl min −1 flow for 2 h, after ethanol is being flowed first (20 μl min −1 for 15 min) and after the modification is finished. The PDMS is removed, the chip is washed again with ethanol for 10 s. The chip is placed on a hot plate at 115 °C for 3 h. OTS monolayers where assembled over dedicated pads beforehand following Sagiv’s method [48] , whereby the cleaned chip is immersed for ca . 30 s in a 5 mM solution of OTS in cyclohexane under controlled environment (25 °C, vapour pressure 50%), followed by sonication for 2 min in toluene. This procedure is repeated once followed by exposing the chip for 12 h to a water saturated atmosphere (100% RH at 40 °C), followed by an additional immersion in the OTS/BCH solution for ca . 30 s, sonication in toluene, and final annealing for 10 min in a preheated oven at 115 °C. This sequence of operations is repeated three times, ending with the thermal annealing at 115 °C. Sensing measurements Qualified devices that ensure good sensor performance, as determined by electrical characterization, were wire-bonded (West- Bond 7476E, Anaheim, CA) to the outer pads of the chip carrier (PCB technologies Ltd Israel. A commercial DC source measure unit (SM32P, FES Israel) enables the simultaneous reading of 64 devices under test. PDMS-molded microfluidic heads supply the pads with alternating control and sensing solutions. The dimensions of the channels dictate a laminar flow with a Pe ~\n200. The fluid is infused or withdrawn by a syringe pump (Mitos XS Dolomite, UK) at a rate of 10–1,000 μl min −1 . XPS measurements XPS studies were performed on SiNWs substrates, using 5,600 Multi-Technique System (PHI, USA) with a base pressure of 2.5 × 10 −10 torr. Samples were irradiated with an Al Kα monochromated source (1486.6 eV) and the out coming electrons were analysed by a Spherical Capacitor Analyzer using a slit aperture of 0.8 mm. Sample charging was compensated (if required) with a charge neutralizer (C1s at 285 eV was taken as an energy reference). The SAM samples were analysed at a shallow take-off angle of 23°. High-resolution XPS measurements were taken at pass energy of 11.75 eV with 0.05 eV per step interval. SiNWs wafers with 600 nm thermal oxide, SSP prime grade, were cut for the XPS studies to 5 × 5 mm 2 pieces. Before the chemical modification, samples were cleaned by an oxygen plasma step, and dehydration on a hot plate for 1–2 h. The different modifications steps were done as described above in the surface functionalization section, except that the chips were immersed in the silane solution for 30 min, washed with ethanol, IPA, ethanol, blown with dry N 2 prior to drying on a hot plate at 115 °C for 3 h (for additional details, see Supplementary Figs 9–15 ). QCM measurements A home-built QCM analyzer equipped with a Fluke 164T multifunction counter was used for the microgravimetric quartz crystal microbalance experiments. Quartz crystals (AT cut, 9 MHz) sandwiched between two Au electrodes (roughness factor ca . 3.5 with an area of 0.196 cm 2 ) were used in microgravimetric experiments, after deposition of a thin silicon oxide layer of 5 nm by PECVD deposition. Quartz electrodes were cleaned with a piranha solution (70% H 2 SO 4 :30% H 2 O 2 ) for 15 min, then rinsed thoroughly with DDW and dried with a stream of argon before chemical modification steps. Thickness measurements by ellipsometry Ellipsometric measurements were carried out on a M-2000DUV Spectroscopic Ellipsometer (J.A.Woollam Co., Inc.). The angles of incidence were 65°, 70° and 75° with a spot size of 2–3 mm. The data were analysed using WVASE32 software installed with the ellipsometer. The film thicknesses of the examined layers were calculated by using the Cauchy model. How to cite this article: Lichtenstein, A. et al . Supersensitive fingerprinting of explosives by chemically modified nanosensors arrays. Nat. Commun. 5:4195 doi: 10.1038/ncomms5195 (2014).